Physical limitations on broadband invisibility based on fast-light media 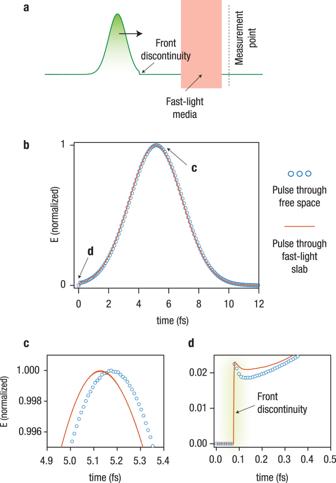Fig. 1: Physical limitations on superluminal pulse propagation due to relativistic causality. aConceptual scheme of a broadband pulse (envelope of a wave packet) propagating through a slab composed of a fast-light medium.bTransmitted electric field envelope, recorded in time using fully causal FDTD simulations, for the pulse propagating through the fast-light medium, superimposed with a companion pulse propagating through free space over the same distance. Zoomed-in view of: (c) the peak of the pulses and (d) their front discontinuities. These illustrative results show that, while the pulse peak can propagate superluminally, the front discontinuity is bounded by the speed of light in vacuum, thus obeying relativistic causality. As discussed in the text, the peak of a smooth pulse does not carry any genuine information that is not already present in the pulse front. As a result, since information cannot travel superluminally, an object cloaked by a three-dimensional fast-light medium, as proposed in Fig. 1. of ref.1, would always be detectable using sufficiently accurate time-of-flight measurements. 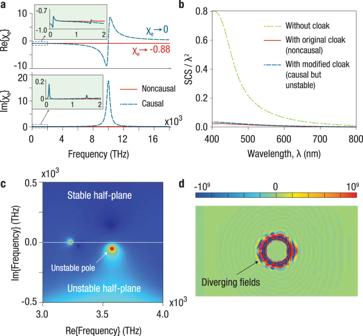Fig. 2: Physical limitations of invisibility cloaks made of fast-light media due to relativistic causality and stability. aElectric susceptibility (top panel, real part; bottom panel, imaginary part) of the original fast-light (gain doublet) cloaking material in Fig. 2 of ref.1(red solid curve) and a modified causal version of this material (blue dashed curve). The material models considered in ref.1violate relativistic causality because the high-frequency limit of the susceptibilities is non-zero and negative. The main panels show the high-frequency limit and the insets show the frequency range of interest for cloaking operation.bNormalized scattering cross section (SCS) based on exact analytical calculations (Mie theory20) for the uncloaked and cloaked spherical dielectric objects considered in Fig. 2 of ref.1. The plot shows the scattering spectra of both the original non-causal cloak, and the modified causal (but unstable) cloak, corresponding, respectively, to the red and blue curves ina.cMagnitude of the scattering coefficient for electric dipole scattering from the causal cloaked sphere, plotted on the complex frequency plane, revealing the presence of an unstable pole.dElectric field distribution (time snapshot of thex-component) around the causal cloaked sphere on thexz-plane. The field profile is shown for a broadband pulse after the pulse has propagated for a duration of 4 fs, clearly showing the diverging fields around the cloaked object due to the onset of unstable (unbounded) oscillations. This implies that the low SCS for the cloaked cases inbis physically irrelevant since the cloaking material is either temporally non-causal or unstable. The scale bar is normalized to the maximum amplitude of the incident wave. Time-domain animation of the field distribution indis given in Supplementary Video1. Simulations All simulations were performed in time-domain via the finite-difference time-domain method using a commercially available software (Lumerical FDTD Solutions). In Fig. 1 , the pulses have a center frequency of 562 THz and a bandwidth of 210 THz. The slab exhibits an average group velocity of 5.5 c 0 over the bandwidth of interest ( c 0 is the velocity of light in vacuum), and has a thickness of 22 nm. In Fig. 2 , the spherical object to be cloaked has a radius of 90 nm and a relative permittivity of 5, while the thickness of the spherical shell cloak is equal to 10 nm. The electric and magnetic susceptibilities of the cloak material follow standard multi-resonator dispersion models, as in Eqs. ( 1 ), ( 2 ), respectively: 
    χ_e(ω )=ε_∞-1+∑_n=1^mf_nω_p1,n^2/ω_0,n^2-ω^2+iωγ_n
 (1) 
    χ_m(ω )=μ_∞-1+∑_n=1^mf_nω_p2,n^2/ω_0,n^2-ω^2+iωγ_n
 (2) The material dispersion parameters of the original “fast-light cloak” (Fig. 2 of ref. [1] , which purportedly included “time-domain simulations snapshots”) are listed below (as provided by the authors through private communications), which correspond to a non-causal gain doublet configuration with two inverted Lorentzian resonances (Fig. 2 a): ε ∞ = 0.12, μ ∞ = 0.06, m = 2, f 1 = f 2 = −1, ω p1,1 = ω p2,1 = 0.05 ω c , ω p1,2 = ω p2,2 = ω c /12, ω 0,1 = 0.25 ω c , ω 0,2 = 3 ω c , γ 1 = γ 2 = 0.06 ω c , ω c = 2 π 500 THz The parameters of our causal dispersion models are listed below, where an additional inverted Lorentzian resonance has been added to both the electric and magnetic susceptibility of the original fast-light material to obtain a causal response (Fig. 2 a). ε ∞ = 1, μ ∞ = 1, m = 3, f 1 = f 2 = f 3 = −1, ω p1,1 = ω p2,1 = 0.05 ω c , ω p1,2 = ω p2,2 = ω c /12, ω p1,3 = 18.762 ω c , ω p2,3 = 19.391 ω c , ω 0,1 = 0.25 ω c , ω 0,2 = 3 ω c , ω 0,3 = 20 ω c , γ 1 = γ 2 = 0.06 ω c , γ 3 = ω c , ω c = 2 π 500 THz The scattering spectra and scattering coefficient in Fig. 2b, c were obtained using exact Mie theory [20] . In Fig. 2d and the Supplementary animation, the pulse has a center frequency of 650 THz and a bandwidth of 500 THz.